Observation and control of Casimir effects in a sphere-plate-sphere system 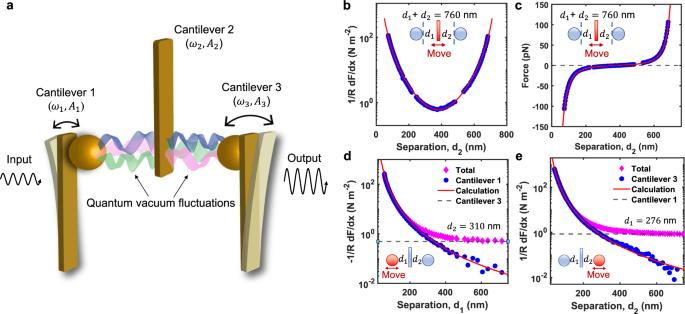Fig. 1: Casimir interaction between three optomechanical resonators. aThree modified cantilevers with resonant frequenciesω1,ω2andω3experience Casimir force between each two nearby surfaces. The vibration amplitudes of three cantilevers are denoted asA1,A2andA3. Additional parametric modulations are applied on the center cantilever to couple them by the Casimir effect. We can switch on and off the Casimir coupling between cantilever 1 and cantilever 3 by controlling the parametric modulations. In addition, we can amplify the energy transfer through Casimir effect by adding an extra gain to cantilever 2.bMeasured Casimir force gradient on cantilever 2 (center) as a function of its position when the other two surfaces are fixed such thatd1+d2= 760 nm. The blue circles are experimental measurements and the red solid line are the theoretical prediction.cThe measured Casimir force on cantilever 2 is shown as a function ofd2.dMeasured Casimir force gradient experienced by cantilever 2 as a function ofd1whend2is fixed at 310 nm. The red diamonds are the total force gradient\(-\frac{1}{R}\frac{dF}{dx}\)measured from cantilever 2. The blue circles are the force gradient contributed from cantilever 1. The red solid curve is the theoretical prediction of the interaction between cantilever 1 and 2. The gray dashed line is the theoretical prediction of the interaction between cantilever 2 and 3 and hence it is independent ofd1under additivity approximation.eMeasured Casimir force gradient on cantilever 2 as a function ofd2whend1is fixed at 276 nm. A remarkable prediction of quantum field theory is that there are quantum electromagnetic fluctuations (virtual photons) everywhere, which leads to the intriguing Casimir effect. While the Casimir force between two objects has been studied extensively for several decades, the Casimir force between three objects has not been measured yet. Here, we report the experimental demonstration of an object under the Casimir force exerted by two other objects simultaneously. Our Casimir system consists of a micrometer-thick cantilever placed in between two microspheres, forming a unique sphere-plate-sphere geometry. We also propose and demonstrate a three-terminal switchable architecture exploiting opto-mechanical Casimir interactions that can lay the foundations of a Casimir transistor. Beyond the paradigm of Casimir forces between two objects in different geometries, our Casimir transistor represents an important development for controlling three-body virtual photon interactions and will have potential applications in sensing and information processing. The interaction between three objects give rise to many fascinating phenomena such as chaos of astronomical objects [1] , Efimov bound states of ultracold atoms [2] , and frustrated states of quantum spin systems [3] . It is intriguing to consider the potential of three-body interactions arising solely from quantum electromagnetic fluctuations (virtual photons) [4] , [5] , [6] . As quantum electromagnetic fluctuations exist everywhere in the universe and in human-made devices, the Casimir effect is ubiquitous. However, the Casimir effect is often neglected or treated as a detrimental effect in micro-electromechanical systems and nano-electromechanical systems [7] . It will be beneficial to develop useful applications of the Casimir effect. One application of the Casimir effect is to provide a new approach to couple mechanical resonators [8] . Different from optomechanical coupling with real photons in cavity optomechanics [9] , [10] , [11] , [12] , optomechanical coupling with virtual photons will not suffer from cavity loss and thus will not require a high-quality cavity. Compared to electrostatic coupling, the Casimir effect does not require charge and will work for both conductors and insulators. Compared to the optical force, the Casimir force works for both transparent and opaque materials. Meanwhile, the use of the Casimir force does not prevent the use of the electrostatic force and the optical force. They may be combined to achieve more advanced functions. In addition, the Casimir effect is energy efficient as it does not require a voltage source or a light source to maintain, which will be particularly important for devices operating in the quantum regime at low temperatures. Recently, the Casimir effect was used to increase the quality factor of a mechanical resonator [13] and couple two separate mechanical resonators [14] , [15] . In addition, the Casimir effect has been utilized to realize nonlinear oscillation [16] , quantum trapping and self-assembling [17] , [18] . While the paradigm of Casimir effect between two objects has been extensively explored [19] , [20] , [21] , [22] , [23] , [24] , [25] , [26] , the Casimir force between three macroscopic objects has not been detected yet. The Casimir effect between three objects will be important in studying gravity at short distances as a metal film is often used to separate two test masses to shield electrostatic interactions [27] , [28] , [29] . Precision measurement of the Casimir effect has been used to search for a new force beyond the standard model [30] . Beyond its fundamental interest, a Casimir system with three objects can open the route to realize crucial technological building blocks such as a transistor-like three-terminal device with quantum vacuum fluctuations. In this article, we report the experimental demonstration of an object under the Casimir force exerted by two other objects simultaneously. We also propose and demonstrate a three-terminal Casimir system that can switch and amplify quantum-vacuum-mediated energy transfer, in analogy to a field effect transistor. Our unique sphere-plate-sphere Casimir system consists of three closely-spaced optomechanical oscillators, as shown in Fig. 1 a. A micrometer-thick cantilever is placed in between two microspheres which are attached to two other cantilevers. Their motions are monitored by three independent fiber-optic interferometers. There are random quantum vacuum fluctuations between them and hence each cantilever experiences a separation-dependent Casimir force. We first measure the Casimir force in this sphere-plate-sphere system. We then apply parametric modulation on cantilever 2 to couple their motion by the Casimir effect. In this way, energy can flow from cantilever 1 to cantilever 2 and to cantilever 3. The center cantilever serves as a gate for controlling the energy transfer through the Casimir effect. By adding gain to the center cantilever with active feedback, we also realize amplification of the quantum-fluctuation-mediated energy transfer. Our Casimir transistor will have promising application in sensing [31] , [32] and information processing [33] , [34] . Fig. 1: Casimir interaction between three optomechanical resonators. a Three modified cantilevers with resonant frequencies ω 1 , ω 2 and ω 3 experience Casimir force between each two nearby surfaces. The vibration amplitudes of three cantilevers are denoted as A 1 , A 2 and A 3 . Additional parametric modulations are applied on the center cantilever to couple them by the Casimir effect. We can switch on and off the Casimir coupling between cantilever 1 and cantilever 3 by controlling the parametric modulations. In addition, we can amplify the energy transfer through Casimir effect by adding an extra gain to cantilever 2. b Measured Casimir force gradient on cantilever 2 (center) as a function of its position when the other two surfaces are fixed such that d 1 + d 2 = 760 nm. The blue circles are experimental measurements and the red solid line are the theoretical prediction. c The measured Casimir force on cantilever 2 is shown as a function of d 2 . d Measured Casimir force gradient experienced by cantilever 2 as a function of d 1 when d 2 is fixed at 310 nm. The red diamonds are the total force gradient \(-\frac{1}{R}\frac{dF}{dx}\) measured from cantilever 2. The blue circles are the force gradient contributed from cantilever 1. The red solid curve is the theoretical prediction of the interaction between cantilever 1 and 2. The gray dashed line is the theoretical prediction of the interaction between cantilever 2 and 3 and hence it is independent of d 1 under additivity approximation. e Measured Casimir force gradient on cantilever 2 as a function of d 2 when d 1 is fixed at 276 nm. Full size image Casimir force in the sphere-plate-sphere configuration We first measure the Casimir force in our sphere-plate-sphere system (Fig. 1 ). Assuming three surfaces are all made of ideal conductive metal and they are sufficiently thick, the Casimir force on the center one is [23] : 
    F_2,C^0=π^3ℏ c/360(R_1/d_1^3-R_2/d_2^3),
 (1) where d 1 and d 2 are the separations between cantilever 1 and cantilever 2, and the separation between cantilever 2 and cantilever 3 as shown in the inset of Fig. 1 b. R 1 and R 2 are the radii of the sphere on cantilever 1 and cantilever 3, respectively. The Casimir force strongly depends on the separations and is highly nonlinear. Such a large nonlinearity is crucial for achieving parametric coupling as described in the next section. The Casimir interaction between real materials can be calculated by the Lifshitz theory [15] , [35] . Our custom Matlab codes to calculate the Casimir interaction in a sphere-plate-sphere system are provided in the Supplementary Software . We use the dynamic force measurement scheme to measure the Casimir force. More details about the calculation of Casimir interaction in our system can be found in Methods and Supplementary Note 1 . The detailed force measurement schemes and results are presented in Supplementary Note 2 and Supplementary Figs. 2 – 5 . The measured Casimir force gradient on cantilever 2 in our three-body system is shown in Fig. 1 b. We fix the position of cantilever 1 and 3 such that d 1 + d 2 = 760 nm. Meanwhile, we change the position of the cantilever 2 (center). As the center cantilever moves from left side to the right side, the gradient meets the lowest value when d 1 = d 2 if R 1 = R 2 . At this specific separation, the net Casimir force on cantilever 2 is zero. The calculation based on Lifshitz’s formula and proximity force approximation is shown in the solid red curve. The measurement is in good agreement with the calculation. We also show the measured Casimir force gradient on cantilever 2 when separation d 1 is changed by moving cantilever 1 in Fig. 1 d, and similarly when separation d 2 is changed by moving cantilever 3 in Fig. 1 e. While there have been many studies of Casimir interaction between two objects, our work reports the measurement of the Casimir force between three separate objects. It opens up the possibility for studying Casimir interaction between more complicated configurations, and can study the nonadditivity nature [36] , [37] , [38] , [39] of the Casimir interaction by reducing the thickness of the center plate (see Supplementary Fig. 1 ). Casimir vibration coupling We now use the Casimir effect to efficiently couple the motions of three cantilevers for realizing a more advanced Casimir-based device. The natural frequencies and damping rates of three cantilevers are ω 1 = 2 π × 5661 Hz, ω 2 = 2 π × 6172 Hz, ω 3 = 2 π × 4892 Hz, γ 1 = 2 π × 3.22 Hz, γ 2 = 2 π × 6.06 Hz, and γ 3 = 2 π × 3.58 Hz when they are far apart. These frequencies shift under Casimir interaction. The direct Casimir coupling strength between three cantilevers is smaller than the frequency differences between them. To solve this issue, we use parametric coupling [15] , [40] by modulating the separation between each two cantilevers at a slow rate ω mod1,2 and a modulation amplitude δ d1,2 . This is achieved by changing the position of the cantilever 2 as \({\delta }_{{{{{{{{\rm{d1}}}}}}}}}\cos ({\omega }_{{{{{{{{\rm{mod1}}}}}}}}}t)+{\delta }_{{{{{{{{\rm{d2}}}}}}}}}\cos ({\omega }_{{{{{{{{\rm{mod2}}}}}}}}}t)\) . Such parametric modulation effectively couples three cantilevers when ω mod1 = ∣ ω 1 − ω 2 ∣ and ω mod2 = ∣ ω 3 − ω 2 ∣ , as shown in Fig. 2 a. Different from direct coupling that requires identical resonant frequencies, parametric coupling provides more freedom to couple different resonators. Under the parametric coupling scheme, the simplified Hamiltonian of the three-cantilever system in the interaction picture is (see Methods and Supplementary Note 4 for detailed derivations) [15] : 
    H=([     -iγ_1/2      g_12/2           0;      g_12/2 -iγ_2/2-δ_2      g_23/2;           0      g_23/2 -iγ_3/2-δ_3 ]). (2) where γ 1,2,3 denote the damping rates of the three cantilevers. \({g}_{12}=\frac{{{{\Lambda }}}_{1}}{2\sqrt{{m}_{1}{m}_{2}{\omega }_{1}{\omega }_{2}}}\) and \({g}_{23}=\frac{{{{\Lambda }}}_{2}}{2\sqrt{{m}_{2}{m}_{3}{\omega }_{2}{\omega }_{3}}}\) are the coupling strengths between cantilever 1 and cantilever 2, and between cantilever 2 and cantilever 3, respectively. Here we have \({{{\Lambda }}}_{1}=\frac{{d}^{2}{F}_{C}}{d{x}^{2}}{|}_{{d}_{10}}{\delta }_{{{{{{{{\rm{d1}}}}}}}}}\) and \({{{\Lambda }}}_{2}=\frac{{d}^{2}{F}_{C}}{d{x}^{2}}{|}_{{d}_{20}}{\delta }_{{{{{{{{\rm{d2}}}}}}}}}\) . Here d 10,20 is the equilibrium separation when there is no modulation applied. δ 2 = ω 1 + ω mod1 − ω 2 and δ 3 = ω 1 + ω mod1 − ω mod2 − ω 3 are the detuning of the system which depend on the modulation frequencies. The eigenvalues of this Hamiltonian near resonant coupling conditions are shown in Fig. 2 b. We can observe a clear two-fold anti-crossing when the detunings δ 3 = δ 2 = 0. Fig. 2: Coupling the vibrations of three cantilevers with the Casimir effect. a Parametric modulation of the Casimir interaction is applied in our system. When ω mod1 = ω 2 − ω 1 , cantilever 1 and cantilever 2 are coupled. Similarly, cantilever 2 and cantilever 3 are coupled when ω mod2 = ω 2 − ω 3 . Here \({\omega }_{{{{{{{{\rm{mod}}}}}}}}1,2}\) is the modulation frequency. b Three eigenvalues of the Hamiltonian in Eq. ( 2 ) as a function of δ 3 when δ 2 = 0 and ∣ g 12 ∣ = ∣ g 23 ∣ = 2 π × 20 Hz. Here δ 2 = ω 1 + ω mod1 − ω 2 and δ 3 = ω 1 + ω mod1 − ω mod2 − ω 3 are the detuning of the system. g 12 and g 23 are the coupling strengths between cantilever 1 and cantilever 2, and between cantilever 2 and cantilever 3, respectively. c Measured power spectrum density (PSD) of cantilever 3 as a function of the modulation frequency ω mod2 . e PSD of cantilever 2 as a function of ω mod2 . The modulation amplitudes are δ d1 = 10.4 nm and δ d2 = 14.1 nm. The modulation frequency ω mod1 is fixed at 440 Hz. d , f The simulated PSD for two cantilevers. The separations are d 10 = 88 nm and d 20 = 90 nm. Full size image Our experimental results of the level repulsion behavior due to the Casimir coupling between three cantilevers are show in Fig. 2 c, e. We study this behavior experimentally by scanning the power spectrum densities (PSD) of cantilever 3 (Fig. 2 c) and cantilever 2 (Fig. 2 e) as a function of the modulation frequency ω mod2 when ω mod1 = ∣ ω 1 − ω 2 ∣ . 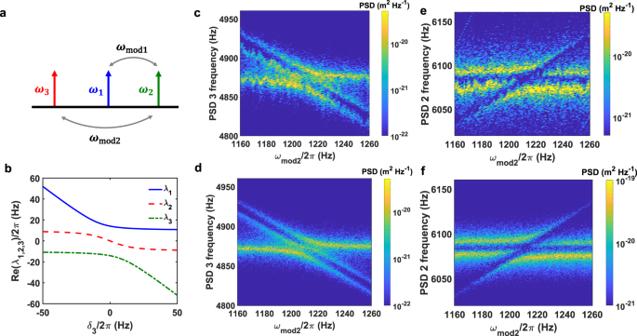Fig. 2: Coupling the vibrations of three cantilevers with the Casimir effect. aParametric modulation of the Casimir interaction is applied in our system. Whenωmod1=ω2−ω1, cantilever 1 and cantilever 2 are coupled. Similarly, cantilever 2 and cantilever 3 are coupled whenωmod2=ω2−ω3. Here\({\omega }_{{{{{{{{\rm{mod}}}}}}}}1,2}\)is the modulation frequency.bThree eigenvalues of the Hamiltonian in Eq. (2) as a function ofδ3whenδ2= 0 and∣g12∣=∣g23∣= 2π× 20 Hz. Hereδ2=ω1+ωmod1−ω2andδ3=ω1+ωmod1−ωmod2−ω3are the detuning of the system.g12andg23are the coupling strengths between cantilever 1 and cantilever 2, and between cantilever 2 and cantilever 3, respectively.cMeasured power spectrum density (PSD) of cantilever 3 as a function of the modulation frequencyωmod2.ePSD of cantilever 2 as a function ofωmod2. The modulation amplitudes areδd1= 10.4 nm andδd2= 14.1 nm. The modulation frequencyωmod1is fixed at 440 Hz.d,fThe simulated PSD for two cantilevers. The separations ared10= 88 nm andd20= 90 nm. Figure 2 e shows three branches which correspond to the hybrid modes of three cantilevers after being projected to cantilever 2. Since ω mod1 is fixed at the resonant value that can couple cantilever 1 and cantilever 2, we notice a clear anti-crossing behavior (a horizontal dark line around 6080 Hz) independent of ω mod2 . The two horizontal branches describe the coupled motion of cantilevers 1 and 2. When we vary ω mod2 , we also observe an inclined branch with a frequency ω 3 + ω mod2 which corresponds to the motion of cantilever 3. When this inclined branch intersects with the other two branches at ω mod2 = ∣ ω 3 − ω 2 ∣ , a more complicated level repulsion is observed. One mode disappears in the PSD of cantilever 2 as this mode only involves the motion of cantilever 1 and 3. More detailed discussions about the eigenvalues and PSD of the system is included in Supplementary Note 4 . Numerical simulation results are shown in Fig. 2 d, f, which agree well with experimental results. Thus we have strongly coupled the motions of three objects with quantum vacuum fluctuations. Casimir switch Our three-terminal Casimir system enables switching (Fig. 3 a) and amplifying quantum-fluctuation-mediated energy transfer in analogy to a field effect transistor (Fig. 3 b). The quantum-fluctuation-mediated energy transfer between cantilever 1 and 3 can be easily switched on and off by controlling the modulation on cantilever 2 (Fig. 3 c). When ω mod1 and ω mod2 are on resonance, vibration energy from cantilever 1 can be transferred to cantilever 3 efficiently (Fig. 3 e). However, when the modulation is off, the excitation on cantilever 1 can not be transferred to cantilever 3 efficiently (Fig. 3 d). In Fig. 3 f, the measured amplitude ratio A 3 / A 1 is shown as a function of modulation frequency ω mod2 for both switch on and off cases. We notice that the amplitude ratio can achieve up to 0.44 when the modulation is on resonance, and close to zero when the modulation if off resonance. Thus we can switch on and off the quantum-fluctuation-mediated energy transfer with high contrast. The separations in Figs. 3 and 4 are larger than those separations in Fig. 2 and give smaller coupling strengths: g 12 = 2 π × 3.5 Hz and g 23 = 2 π × 3.9 Hz. These coupling strengths are comparable to the damping rates of the cantilevers so there is no mode splitting in this case. Fig. 3: Switching quantum-fluctuation-mediated energy transfer. a A symbolic switch. b A symbolic field effect transistor. c The quantum-fluctuation-mediated energy transfer between cantilever 1 and 3 can be switched on and off by the modulation on cantilever 2. The position of cantilever 2 is modulated with modulation amplitudes δ d1,2 and modulation frequencies ω mod1,2 . d Measured displacement of two cantilevers ( x 1 and x 3 ) when modulation is off. e Measured displacement of two cantilevers when modulation is on. Energy from cantilever 1 is transferred efficiently to cantilever 3. Here ω mod1,2 = 2 π × 465 Hz, ω mod2 = 2 π × 1230 Hz, δ d1 = 6.0 nm, and δ d2 = 8.5 nm. The separations are d 10 = 100 nm and d 20 = 105 nm. f The transduction ratio A 3 / A 1 is shown as a function of the modulation frequency ω mod2 when ω mod1 is on resonant. A 1 and A 3 are the vibrational amplitudes. The blue circles and the red diamonds correspond to the switch on and off case, respectively. The magenta solid line is the simulation. g The transduction ratio A 3 / A 1 as a function of modulation amplitude δ d1 when ω mod2 = 2 π × 1231 Hz (on resonant, blue circles) and ω mod2 = 2 π × 1150 Hz (off resonant, red diamonds). ω mod1 is on resonant for both cases. The magenta solid curve is the simulation and the green solid curve is the calculation based on Eq. ( 3 ). Full size image Fig. 4: Amplifying quantum-fluctuation-mediated energy transfer. a An extra gain G is applied on cantilever 2 by feedback control together with parametric modulation. b The signal on cantilever 1 ( x 1 ) is transmitted to cantilever 3 ( x 3 ) with amplification. c The transduction ratio A 3 / A 1 is shown as a function of modulation frequency ω mod2 when the gain is on (red diamonds) and off (blue circles). ω mod1 is on resonant for both cases. G is the gain coefficient on cantilever 2. Under the extra gain, the damping rate of cantilever 2 becomes γ 2 = γ 20 − G , where γ 20 is the natural damping rate. The cyan and magenta solid curve are the simulations. 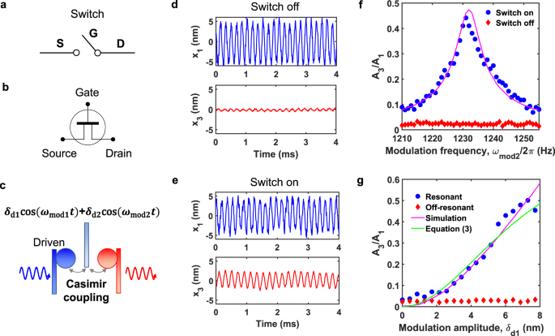Fig. 3: Switching quantum-fluctuation-mediated energy transfer. aA symbolic switch.bA symbolic field effect transistor.cThe quantum-fluctuation-mediated energy transfer between cantilever 1 and 3 can be switched on and off by the modulation on cantilever 2. The position of cantilever 2 is modulated with modulation amplitudesδd1,2and modulation frequenciesωmod1,2.dMeasured displacement of two cantilevers (x1andx3) when modulation is off.eMeasured displacement of two cantilevers when modulation is on. Energy from cantilever 1 is transferred efficiently to cantilever 3. Hereωmod1,2= 2π× 465 Hz,ωmod2= 2π× 1230 Hz,δd1= 6.0 nm, andδd2= 8.5 nm. The separations ared10= 100 nm andd20= 105 nm.fThe transduction ratioA3/A1is shown as a function of the modulation frequencyωmod2whenωmod1is on resonant.A1andA3are the vibrational amplitudes. The blue circles and the red diamonds correspond to the switch on and off case, respectively. The magenta solid line is the simulation.gThe transduction ratioA3/A1as a function of modulation amplitudeδd1whenωmod2= 2π× 1231 Hz (on resonant, blue circles) andωmod2= 2π× 1150 Hz (off resonant, red diamonds).ωmod1is on resonant for both cases. The magenta solid curve is the simulation and the green solid curve is the calculation based on Eq. (3). d The vibrational amplitude A 3 is shown as a function of amplitude A 1 for three different gain coefficients G . The parametric modulation is applied resonantly at the same time. The green, magenta and blue solid line are the simulated results for three different gain coefficients. e The ratio A 3 / A 1 is shown as a function of modulation amplitude δ d1 for cases with gain, no gain, and off-resonant modulation. δ d2 = 1.42 δ d1 . f The transduction ratio A 3 / A 1 (blue circles) is shown as a function of the extra feedback gain G applied on cantilever 2. The red solid curve is the simulation. Full size image Under the steady state when the cantilever 1 is driven at ω 1 with a small amplitude and the parametric modulation on cantilever 2 is on resonant, the transduction ratio A 3 / A 1 in this three-cantilever Casimir system is (see Methods): 
    A_3/A_1=|Λ_1Λ_2/4m_2m_3ω_2ω_3γ_2γ_3+Λ_2^2|. (3) where \({{{\Lambda }}}_{1}=\frac{{d}^{2}{F}_{C}}{d{x}^{2}}{|}_{{d}_{10}}{\delta }_{{{{{{{{\rm{d1}}}}}}}}}\) and \({{{\Lambda }}}_{2}=\frac{{d}^{2}{F}_{C}}{d{x}^{2}}{|}_{{d}_{20}}{\delta }_{{{{{{{{\rm{d2}}}}}}}}}\) . For Fig. 3 , the cantilever 1 is driven at 5649 Hz, which is its resonant frequency in this situation. In Fig. 3 g, the measured transduction ratio A 3 / A 1 is shown as a function of modulation amplitude δ d1 when δ d2 = 1.42 δ d1 . The transduction ratio is close to zero when the parametric modulation is off-resonant. As expected, the ratio A 3 / A 1 increases when δ d1 increases under resonant coupling. Our experimental results agree well with Eq. ( 3 ) and numerical simulation results (Fig. 3 g). Casimir amplification To realize a Casimir transistor with high efficiency, we introduce an extra gain to the system (Fig. 4 a) to amplify the quantum-fluctuation-mediated energy transfer. The extra gain is applied to cantilever 2 by feedback control such that the damping rate of cantilever 2 becomes γ 2 = γ 20 − G , where γ 20 is the natural damping rate of cantilever 2 and G is the gain coefficient (More details can be found in Supplementary Note 3 and Supplementary Fig. 6 ). γ 2 becomes negative when G > γ 20 . Based on Eq. ( 3 ), the transduction ratio A 3 / A 1 increases when γ 2 decreases. Under such condition, energy from cantilever 1 is first transferred to cantilever 2 and get amplified and then transferred to cantilever 3. For example, we apply a fixed gain to cantilever 2 such that G = 2 π × 8.73 Hz to realize the amplification of energy transfer, as shown in Fig. 4 b. Other parameters are the same as those in Fig. 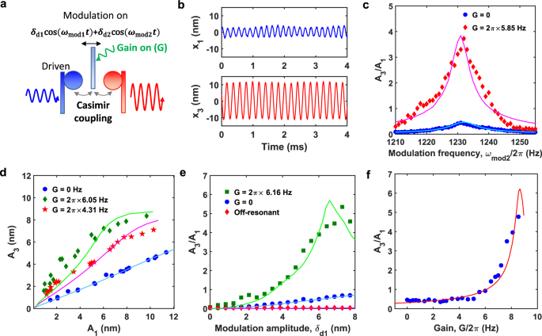Fig. 4: Amplifying quantum-fluctuation-mediated energy transfer. aAn extra gainGis applied on cantilever 2 by feedback control together with parametric modulation.bThe signal on cantilever 1 (x1) is transmitted to cantilever 3 (x3) with amplification.cThe transduction ratioA3/A1is shown as a function of modulation frequencyωmod2when the gain is on (red diamonds) and off (blue circles).ωmod1is on resonant for both cases.Gis the gain coefficient on cantilever 2. Under the extra gain, the damping rate of cantilever 2 becomesγ2=γ20−G, whereγ20is the natural damping rate. The cyan and magenta solid curve are the simulations.dThe vibrational amplitudeA3is shown as a function of amplitudeA1for three different gain coefficientsG. The parametric modulation is applied resonantly at the same time. The green, magenta and blue solid line are the simulated results for three different gain coefficients.eThe ratioA3/A1is shown as a function of modulation amplitudeδd1for cases with gain, no gain, and off-resonant modulation.δd2= 1.42δd1.fThe transduction ratioA3/A1(blue circles) is shown as a function of the extra feedback gainGapplied on cantilever 2. The red solid curve is the simulation. 3 e. Figure 4 c shows amplification of quantum-fluctuation-mediated energy transfer with our Casimir transistor. When a gain is applied to cantilever 2, energy transfer from cantilever 1 to cantilever 3 shows a similar resonant behavior as the no-gain case, but has an improvement by a factor of 8 on the transduction ratio . The additional gain improves the quantum-fluctuation-mediated energy transfer efficiency significantly. As expected, the transduction ratio A 3 / A 1 increases when the parametric modulation amplitude (Fig. 4 e) or the gain coefficient (Fig. 4 d, f) increases until the system becomes unstable when the modulation amplitude or the gain is too large. Thus we have demonstrated amplification in a three-terminal Casimir system. The amplification function will be crucial for future applications of Casimir-based devices. For example, Casimir parametric amplification has been theoretically proposed for zeptometer metrology [31] and ultrasensitive magnetic gradiometry [32] . We have measured the Casimir interaction between three objects, and demonstrated efficient coupling of three optomechanical resonators with virtual photons. Compared to the conventional optomechanical coupling with real photons in a high-Q cavity [9] , [10] , optomechanical coupling with virtual photons [8] , [41] does not need a high-Q cavity. Inspired by a field effect transistor, we also demonstrate switching and amplifying quantum-fluctuation-mediated energy transfer in our three-terminal Casimir system. As proposed by former theoretical studies, Casimir-based amplification and switching will have applications in sensing [31] , [32] and information processing [33] , [34] . The realization of Casimir coupling between three resonators is an important step toward realizing a scalable Casimir array. The three resonators can also be modified to realize a circulator in the future, which can have non-reciprocity between any two of the three resonators [42] . By reducing the thickness of the center cantilever, the system can be used to study non-pairwise additive effects [38] , [39] . The Casimir effect between three objects is also important in studying gravity at short distances [27] , [28] , [29] . Casimir force calculation At a finite temperature, the Casimir interaction comes from both quantum and thermal fluctuations. At temperature T and separation x , the Casimir energy per unit area between two surfaces is given by [35] : 
    [ E(x,T)=k_BT/2π∑_l=0^∞^'∫_0^∞k_⊥dk_⊥{ln [1-r_TM^2(iξ_l,k_⊥)e^-2xq]+ln [1-r_TE^2(iξ_l,k_⊥)e^-2xq]}, ]
 (4) where \({\xi }_{l}=\frac{2\pi {k}_{B}Tl}{\hslash }\) is the Matsubara frequency and \({k}_{\perp }=\sqrt{{k}_{x}^{2}+{k}_{y}^{2}}\) is the wave vector parallel to the surface. r T E ( i ξ l , k ⊥ ) and r T M ( i ξ l , k ⊥ ) are reflection coefficients of the transverse-electric and transverse-magnetic modes. The separation between two surfaces is far smaller than the dimensions of the cantilever and the sphere. Therefore, we can apply the proximity-force approximation and the Casimir force between a sphere with radius R and a plate is F C ( x , T ) = − 2 π R E ( x , T ). The calculation in ref. 15 has shown that the contribution from thermal fluctuations at room temperature is less than 4% when the separation is less than 800 nm. Thus, the Casimir interaction in our system is dominated by quantum vacuum fluctuations. In our system, the thickness of the center cantilever is 1 μm and the typical separation in our measurement is from 50 to 800 nm. Under such condition, the contribution from the nonadditivity is negligible compared to the sum of the pair potential and hence we take the additivity approximation [36] . Under the thermal equilibrium, the force on the center cantilever can be simplified as F 2, C = − F C ( d 1 , T ) + F C ( d 2 , T ). Under the additivity approximation, the force gradient between cantilever 1 and cantilever 2 is calculated by subtracting the force gradient between cantilever 2 and cantilever 3 from the total gradient experienced by cantilever 2, as shown in Fig. 1 d. Experimental setup and force measurement In the experiment, we use three modified AFM cantilevers to build the three-terminal Casimir system. The left and right cantilever has a dimension of 450 × 50 × 2 μm 3 . The center cantilever has a dimension of 500 × 100 × 1 μm 3 . Two 70-μm-diameter polystyrene spheres are attached to the free end of the left and right cantilevers to create the sphere-plate-sphere geometry. Additional 100-nm-thick gold layers are coated on both the sphere and cantilever surfaces. During the measurement, we use phase-lock loop to track the resonant frequency in the presence of the Casimir interaction. Then we can get the force gradient as \(\frac{dF}{dx}=-2k\frac{\delta \omega }{\omega }\) , where k is the spring constant of the cantilever, δ ω is the frequency shift in the presence of the interaction and ω is the natural resonant frequency. The separation between each two surfaces is calibrated by the electrostatic force. The frequency shift due to the electrostatic force and the Casimir force is \({{\Delta }}\omega=-\frac{\omega }{2k}\frac{\pi {\epsilon }_{0}R}{{x}^{2}}[{({V}_{{{{{{{{\rm{ext}}}}}}}}}-{V}_{{{{{{{{\rm{c}}}}}}}}})}^{2}+{V}_{{{{{{{{\rm{rms}}}}}}}}}^{2}]-\frac{\omega }{2k}\frac{d{F}_{C}}{dx}\) , where V ext is the external voltage applied on the surface, V c is the patch potential, V rms is the rms voltage fluctuations. \(\frac{d{F}_{C}}{dx}\) is the force gradient of the Casimir interaction at separation x . By measuring the frequency shift of the cantilever for different external voltage V ext , we can calculate the real separation between two surfaces. Our measurements show that the contribution from the rms voltage fluctuations is negligible compared to the Casimir force. After canceling the contribution from electrostatic force, we can get the Casimir force gradient. The Casimir force gradient can be integrated over separation to obtain the Casimir force. Casimir force coupling and energy transfer Under a slow modulation on cantilever 2, the separation between each two cantilevers is time-dependent such that: 
    d_1(t)=	d_10-δ_d1cos (ω_mod1t)-δ_d2cos (ω_mod2t)
     	+x_1(t)-x_2(t),
    d_2(t)=	d_20+δ_d1cos (ω_mod1t)+δ_d2cos (ω_mod2t)
     	+x_2(t)-x_3(t). (5) Here d 10,20 is the equilibrium separation when there is no modulation applied, δ d1,d2 is the modulation amplitude, and ω mod1,2 are two modulation frequencies. x 1 ( t ), x 2 ( t ) and x 3 ( t ) describe vibrations of three cantilevers near their equilibrium positions. The motions of the cantilevers follow equations: 
    m_1ẍ_̈1̈+m_1γ_1ẋ_̇1̇+m_1ω_1^2x_1=	 F_C(d_1(t))
    m_2ẍ_̈2̈+m_2γ_2ẋ_̇2̇+m_2ω_2^2x_2=	 -F_C(d_1(t))+F_C(d_2(t))
    m_3ẍ_̈3̈+m_3γ_3ẋ_̇3̇+m_3ω_3^2x_3=	 -F_C(d_2(t))
 (6) Here we generalize the displacements x 1,2,3 ( t ) to complex values z 1,2,3 ( t ) such that x 1,2,3 ( t ) = R e [ z 1,2,3 ( t )]. We separate the fast-rotating term and the slow-varying term for z 1,2,3 ( t ) such that: 
    z_1,2,3(t)=B_1,2,3(t)e^-iω_1,2,3t,
 (7) where B 1,2,3 ( t ) is the slow-varying amplitudes and we can neglect their second derivative terms \({\ddot{B}}_{1,2,3}(t)\) in the equations of motion. Under the limit of the small damping rate of three cantilevers such that γ 1,2,3 ≪ ω 1,2,3 and the rotating wave approximation, the equation of motion can written as: 
    i([ Ḃ_̇1̇^̇'̇(t); Ḃ_̇2̇^̇'̇(t); Ḃ_̇3̇^̇'̇(t) ])=([     -iγ_1/2 Λ_1/4m_1ω_1           0; Λ_1/4m_2ω_2 -iγ_2/2-δ_2 Λ_2/4m_2ω_2;           0 Λ_2/4m_3ω_3 -iγ_3/2-δ_3 ])([ B_1^'(t); B_2^'(t); B_3^'(t) ]),
 (8) where \({{{\Lambda }}}_{1,2}=\frac{{d}^{2}{F}_{C}}{d{x}^{2}}{|}_{{d}_{10,20}}{\delta }_{{{{{{{{\rm{d1,2}}}}}}}}}\) . We have applied the transformation such that \({B}_{1}^{\prime}(t)={B}_{1}(t)\) , \({B}_{2}^{\prime}(t)={B}_{2}(t){e}^{i{\delta }_{2}t}\) , and \({B}_{3}^{\prime}(t)={B}_{3}(t){e}^{i{\delta }_{3}t}\) , where δ 2 = ω 1 + ω mod1 − ω 2 and δ 3 = ω 1 + ω mod1 − ω mod2 − ω 3 are the system detunings. Under the steady condition, \({\dot{B}}_{1}\) , \({\dot{B}}_{2}\) , and \({\dot{B}}_{3}\) all equal to zero. The vibration amplitude of three cantilevers A 1,2,3 is the absolute value of the slow-varying component so we have A 1,2,3 ( t ) = ∣ B 1,2,3 ( t ) ∣ . In this way, the ratio of A 3 / A 1 is: 
    A_3/A_1=|B_3/B_1|=|Λ_1Λ_2/4m_2m_3ω_2ω_3γ_2γ_3+Λ_2^2|. (9) The vibrations of the three cantilevers can be quantized as phonons. By introducing normalized amplitudes \({c}_{1}=\sqrt{\frac{{m}_{1}{\omega }_{1}}{\hslash }}{B}_{1}^{\prime}\) , \({c}_{2}=\sqrt{\frac{{m}_{2}{\omega }_{2}}{\hslash }}{B}_{2}^{\prime}\) , and \({c}_{3}=\sqrt{\frac{{m}_{3}{\omega }_{3}}{\hslash }}{B}_{3}^{\prime}\) , we obtain the equation of motion for the phonon modes as: 
    i([ ċ_̇1̇; ċ_̇2̇; ċ_̇3̇ ])=([     -iγ_1/2      g_12/2           0;      g_12/2 -iγ_2/2-δ_2      g_23/2;           0      g_23/2 -iγ_3/2-δ_3 ])([ c_1; c_2; c_3 ]),
 (10) where \({g}_{12}=\frac{{{{\Lambda }}}_{1}}{2\sqrt{{m}_{1}{m}_{2}{\omega }_{1}{\omega }_{2}}}=\frac{{d}^{2}{F}_{C}}{d{x}^{2}}{|}_{{d}_{10}}{\delta }_{{{{{{{{\rm{d1}}}}}}}}}\frac{1}{2\sqrt{{m}_{1}{m}_{2}{\omega }_{1}{\omega }_{2}}}\) , and \({g}_{23}=\frac{{{{\Lambda }}}_{2}}{2\sqrt{{m}_{2}{m}_{3}{\omega }_{2}{\omega }_{3}}}=\frac{{d}^{2}{F}_{C}}{d{x}^{2}}{|}_{{d}_{20}}{\delta }_{{{{{{{{\rm{d2}}}}}}}}}\frac{1}{2\sqrt{{m}_{2}{m}_{3}{\omega }_{2}{\omega }_{3}}}\) . Here we consider a special case that g 12 = g 23 , γ 1 = γ 3 , and δ 2,3 = 0. The eigenvalues of the Hamiltonian are: 
    λ_1=	 -iγ_1/2,
    λ_2=	 -iγ_1+γ_2/4+√(8g_12^2-(γ_1-γ_2)^2)/4,
    λ_3=	 -iγ_1+γ_2/4-√(8g_12^2-(γ_1-γ_2)^2)/4. (11) When the coupling strength is large compared to the damping difference such that \(|{g}_{12}|\, > \, \frac{|{\gamma }_{1}-{\gamma }_{2}|}{2\sqrt{2}}\) , we have \({{\rm{Im}}}({\lambda }_{2})=-\frac{{\gamma }_{1}+{\gamma }_{2}}{4}\) and hence the steady state requires that: 
    γ_1+γ_2  >   0. (12) When the coupling strength is small compared to damping difference such that \(|{g}_{12}| < \frac{|{\gamma }_{1}-{\gamma }_{2}|}{2\sqrt{2}}\) , we have \({{\rm{Im}}}({\lambda }_{2})=-\frac{{\gamma }_{1}+{\gamma }_{2}}{4}+\frac{\sqrt{{({\gamma }_{1}-{\gamma }_{2})}^{2}-8{g}_{12}^{2}}}{4}\) . The steady state requires that: 
    γ_1+γ_2-√((γ_1-γ_2)^2-8g_12^2)  >   0. (13)